Hopping transport through defect-induced localized states in molybdenum disulphide Molybdenum disulphide is a novel two-dimensional semiconductor with potential applications in electronic and optoelectronic devices. However, the nature of charge transport in back-gated devices still remains elusive as they show much lower mobility than theoretical calculations and native n-type doping. Here we report a study of transport in few-layer molybdenum disulphide, together with transmission electron microscopy and density functional theory. We provide direct evidence that sulphur vacancies exist in molybdenum disulphide, introducing localized donor states inside the bandgap. Under low carrier densities, the transport exhibits nearest-neighbour hopping at high temperatures and variable-range hopping at low temperatures, which can be well explained under Mott formalism. We suggest that the low-carrier-density transport is dominated by hopping via these localized gap states. Our study reveals the important role of short-range surface defects in tailoring the properties and device applications of molybdenum disulphide. Layered transition metal dichalcogenide is an emerging class of two-dimensional (2D) materials with attractive electronic and optical properties [1] , [2] , [3] . Among them, molybdenum disulphide (MoS 2 ) is a semiconductor with bandgap of ~1.1–2 eV (refs 4 , 5 ), which is more suitable than graphene for complementary-metal-oxide-semiconductor (CMOS)-like logic device applications. The true 2D nature makes MoS 2 outperform Si transistors at the scaling limit [6] , [7] . Recently, many MoS 2 -based devices have been demonstrated, including field-effect transistors [8] , [9] , [10] , integrated circuits [11] and photo transistors [12] . Gate-tunable metal–insulator transition and superconductivity have been observed in MoS 2 (ref. 13 ). Despite the rapid progress in MoS 2 device applications, the nature of charge transport still remains elusive. In particular, the mobility of back-gated few-layer MoS 2 (meaning 1–3 layers in the rest of the paper) devices was usually over an order of magnitude lower than the theoretical limit set by phonon scattering [8] , [10] , [11] , [14] , [15] . These devices exhibit insulating behaviour at low carrier densities [10] , [13] , [16] . Several possible scattering mechanisms have been proposed including phonons [15] , [17] , Coulomb impurities [8] , [18] and short-range disorder such as interfacial bonding/roughness [19] , yet the nature of the disorders remains to be unequivocally identified. On the other hand, the conductivity of few-layer MoS 2 is extremely sensitive to ambient environments [10] , [20] , indicating an important role of surface defects in charge transport. In addition, the origin of n-type doing in few-layer MoS 2 devices is still unclear. In this work, we combine variable-temperature transport measurements, aberration-corrected transmission electron microscopy (TEM), density functional theory (DFT) and tight-binding calculations to investigate the nature of charge transport in few-layer MoS 2 . We observe sulphur vacancies (SVs) on the surface of MoS 2 , which act as electron donors and induce localized states in the bandgap. Below a critical carrier density, electrons are localized and transport is dominated by nearest-neighbour hopping and variable-range hopping (VRH) at high and low temperatures, respectively. The experimental data can be well explained under Mott’s formalism. Our model suggests a microscopic picture of metal–insulator transition and n-type doping observed in MoS 2 samples. Finally, we discuss the effect of screening and thickness on the charge transport of MoS 2 . Device fabrication and transport measurement The back-gated few-layer MoS 2 devices were fabricated on 300 nm SiO 2 /Si substrate as described in our previous work [10] (see Methods). We have measured 15 samples, all of which showed the same qualitative behaviour. 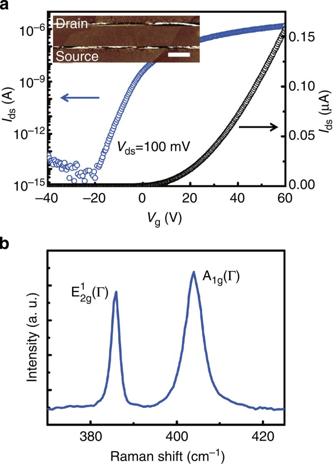Figure 1: Electrical and Raman data. (a)Ids–Vgcharacteristics of a back-gated single-layer MoS2device in both linear and log scale underVds=100 mV. Inset is an atomic force microscopy image of the device, scale bar, 2 μm. (b) Raman spectroscopy using a 514-nm laser on the device to confirm single-layer. Figure 1a shows the room temperature transfer ( I ds –V g ) characteristics of the single-layer MoS 2 device after vacuum annealing at 350 K. The single-layer nature was confirmed by the position and relative intensity of the zone-centre mode (385.9 cm −1 ) and mode (404 cm −1 ) in Raman spectroscopy [21] ( Fig. 1b ). The device exhibited an n-type transistor behaviour with on/off ratio over 10 8 and a field-effect mobility of 7.7 cm 2 V −1 s −1 , which was comparable to the mobility of back-gated devices made similarly. The mobility of the same device measured in ambient was 0.57 cm 2 V −1 s −1 due to oxygen and water absorption [10] . Figure 1: Electrical and Raman data. ( a ) I ds –V g characteristics of a back-gated single-layer MoS 2 device in both linear and log scale under V ds =100 mV. Inset is an atomic force microscopy image of the device, scale bar, 2 μm. ( b ) Raman spectroscopy using a 514-nm laser on the device to confirm single-layer. Full size image We measured the conductivity as a function of carrier density n=C g (V g –V th ) in a cryogenic probe station from room temperature down to ~20 K, where C g =1.15 × 10 −4 Fm −2 is the gate capacitance and V th is the threshold voltage extracted by linear extrapolation of I ds –V ds characteristics in the linear region ( Fig. 1a ). We focused our attention on low-density regimes up to ~3 × 10 12 cm −2 , much lower than that achieved using ionic liquid gate [9] , [13] . Insulating behaviour was observed throughout the whole temperature and carrier density range [16] , which ruled out phonons as the dominant scattering source. 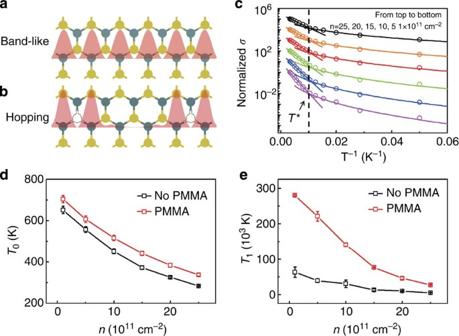Figure 2: Electron hopping transport in MoS2. Schematics of electron transport mechanism in perfect (a) and defective (b) MoS2. In perfect MoS2, electron density is periodic in space and transport is band-like. In defective MoS2, however, electrons are localized near the defects and transport is through hopping. (c) Arrhenius plot of normalized conductivity (symbols) of the device inFig. 1and the fitting results by hopping model (lines). From top to bottom,n=25, 20, 15, 10, 5, 1 × 1011cm−2, respectively. The curves are offset for clarity. The two hopping regimes are clearly separated byT*(dashed vertical line). (d)T0and (e)T1obtained from the fitting of the Arrhenius plot for bare (black) and PMMA-coated (red) sample. The Arrhenius plot after PMMA coating is presented inSupplementary Fig. S10. Figure 2c shows the Arrhenius plot of the normalized conductivity σ under various n . The charge transport exhibited two distinct scaling behaviour at high and low temperature regimes, separated by a characteristic temperature T * on the order of 100 K. At T>T * , the transport was activated, which could not be explained by the Schottky barrier at the contacts but rather came from the channel [16] , as T 0 was an order of magnitude smaller than the expected barrier height (>0.33 eV) considering the work function of Ti contacts and electron affinity of MoS 2 (ref. 22 ). At T<T * , σ transformed to a much weaker temperature dependence that could be fitted very well by the 2D VRH equation Figure 2: Electron hopping transport in MoS 2 . Schematics of electron transport mechanism in perfect ( a ) and defective ( b ) MoS 2 . In perfect MoS 2 , electron density is periodic in space and transport is band-like. In defective MoS 2 , however, electrons are localized near the defects and transport is through hopping. ( c ) Arrhenius plot of normalized conductivity (symbols) of the device in Fig. 1 and the fitting results by hopping model (lines). From top to bottom, n =25, 20, 15, 10, 5, 1 × 10 11 cm −2 , respectively. The curves are offset for clarity. The two hopping regimes are clearly separated by T * (dashed vertical line). ( d ) T 0 and ( e ) T 1 obtained from the fitting of the Arrhenius plot for bare (black) and PMMA-coated (red) sample. The Arrhenius plot after PMMA coating is presented in Supplementary Fig. S10 . Full size image Such characteristic temperature dependence has been observed in many low-dimensional systems and is a signature of hopping transport via localized states [23] , [24] . The localized states and low mobility are not likely introduced by long-range Coulomb impurities from the SiO 2 substrate. The mobility of graphene on similar SiO 2 substrates is limited by Coulomb effect to be ~10 4 cm 2 V −1 s −1 (refs 25 , 26 ), much higher than the intrinsic MoS 2 mobility limit. Another possibility is the chemical bonding to SiO 2 (ref. 19 ), which lacks direct evidence. In addition, such chemical bonding would require dangling bonds in MoS 2 , most probably associated with structural defects. In light of the TEM characterizations below, we attribute the localized states to short-range structural disorders in MoS 2 . TEM characterization To reveal nature of the disorders, we transferred the exfoliated MoS 2 samples to TEM grids and performed aberration-corrected TEM characterizations under 80 keV acceleration voltage (see Methods). A typical atomic image of a single-layer MoS 2 showed the expected hexagonal symmetry but with a high density of defects as bright spots in position of sulphur atoms ( Fig. 3a , red arrows). The defects can be clearly distinguished by analysing the intensity profile. 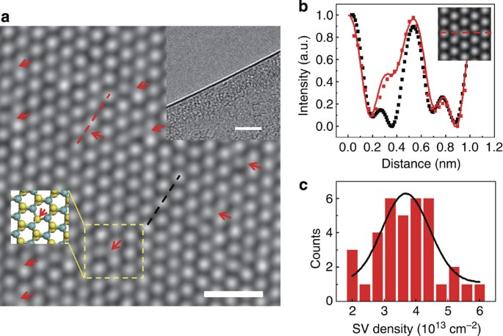Figure 3: TEM of MoS2showing evidence of SVs. (a) Atomic structures of a single-layer MoS2by aberration-corrected TEM. The SVs are highlighted by red arrows. Upper inset shows the MoS2sample edge to confirm the single-layer nature. Lower inset shows the schematics of the highlighted region. Scale bar, 10 nm. (b) Intensity profile of along lattices with (red symbol) and without (black symbol) SV, along with simulations of a single SV (red line). The corresponding sections are highlighted inaby dashed lines. Inset shows the simulated TEM image of a single SV. (c) Histogram of SV density. The density was obtained by counting the number of SVs in 5 × 5 nm2areas. Comparison between intensity profiles along the red dashed line in Figure 3a and simulated high-resolution TEM image of single SV [27] shows quantitative agreement ( Fig. 3b ), which confirms that most defects are single SV. Statistical analysis on more than 30 areas from three samples showed the density of SV on the order of 10 13 cm −2 ( Fig. 3c ), corresponding to an average defect distance a ~1.7 nm. We also observed other point or line defects, but with much lower density. Figure 3: TEM of MoS 2 showing evidence of SVs. ( a ) Atomic structures of a single-layer MoS 2 by aberration-corrected TEM. The SVs are highlighted by red arrows. Upper inset shows the MoS 2 sample edge to confirm the single-layer nature. Lower inset shows the schematics of the highlighted region. Scale bar, 10 nm. ( b ) Intensity profile of along lattices with (red symbol) and without (black symbol) SV, along with simulations of a single SV (red line). The corresponding sections are highlighted in a by dashed lines. Inset shows the simulated TEM image of a single SV. ( c ) Histogram of SV density. The density was obtained by counting the number of SVs in 5 × 5 nm 2 areas. Full size image Great care was taken in TEM experiments to prevent knock-on damage or lattice reconstruction caused by 80 keV electron beam irradiation [28] , [29] . To rule out the effect of electron irradiation on vacancy density, we studied the evolution of defects under different exposure time. As shown in Supplementary Fig. S1 , we did not observe significant number of new SV after 44 s exposure. The vacancy number increased from 65 to 70 in a 12 × 12 nm monolayer MoS 2 area after 62 s exposure. The average vacancy generation rate was 5.6 × 10 10 cm −2 s −1 , which was in a reasonable agreement with the value of 3.8 × 10 10 cm −2 s −1 in ref. 29 . The estimate of vacancy density introduced by electron irradiation during imaging was ~10 12 cm −2 , which was far less than the statistical results shown in Fig. 3c . We thus concluded that the SVs were intrinsic rather than introduced by electron beam irradiation. After hundreds of seconds of irradiation, we started to observe line defects, nanopores or even non-stoichiometric structure in MoS 2 (see Supplementary Fig. S2 ); however, those defects were irrelevant to the current work. DFT calculation The SV causes unsaturated electrons in the surrounding Mo atoms and acts as electron donors to make the MoS 2 electron rich as experimentally observed [8] , [10] , [11] , [13] , [16] . To understand the implication of SV to the band structure of MoS 2 , we performed the DFT calculations on a 5 × 5 single-layer MoS 2 supercell with a single SV ( Fig. 4a , see Methods), corresponding to a SV density of ~4.6 × 10 13 cm −2 . The defect-free MoS 2 has a direct bandgap of 1.67 eV, consistent with earlier DFT calculations [30] and experiments [4] , [5] . The presence of the SV introduces defect states in the bandgap and leads to a transition from direct to indirect 1.61 eV bandgap. The gap state is a deep donor state (0.46 eV below conduction band minimum) and is composed of two individual states, which are degenerate at Γ point but separated by 14 meV at M point ( Fig. 4a ). The bottom of the conduction band is dominated by Mo 4d orbitals, showing a strong degree of delocalization (see Supplementary Fig. S3 ). On the contrary, the gap state and top of valence band are the results of hybridization between strong Mo 4d orbitals and weak S 3p orbitals. The nearly dispersionless midgap state indicates a high electron mass and strong localization near the five-fold Mo atoms surrounding the SV, which is evident from the spatial mapping of these states ( Fig. 4c inset). The electrons are mainly distributed within 3 Å radius surrounding the SV ( Fig. 4c ). In contrast, electrons in the valance band of perfect MoS 2 are delocalized. 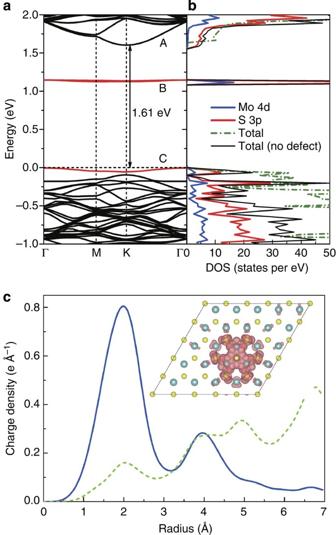Figure 4: DFT calculations. Band structure (a) and partial density of states (b) for single-layer MoS25 × 5 supercell with an SV (seeSupplementary Fig. S4for the supercell structure). The localized states are highlighted by red lines. Green dashed line corresponds to the case without SV. (c) Blue solid line, radial distribution of charge density for the localized midgap state (B and B) ina; green dashed line, radial distribution of charge density for the delocalized top of valance band in perfect MoS2. The origin is located at the SV. Inset is the isosurface (ρ=7 × 10−3e Å−3) of the decomposed charge density corresponding to the band B ina. Figure 4: DFT calculations. Band structure ( a ) and partial density of states ( b ) for single-layer MoS 2 5 × 5 supercell with an SV (see Supplementary Fig. S4 for the supercell structure). The localized states are highlighted by red lines. Green dashed line corresponds to the case without SV. ( c ) Blue solid line, radial distribution of charge density for the localized midgap state (B and B) in a ; green dashed line, radial distribution of charge density for the delocalized top of valance band in perfect MoS 2 . The origin is located at the SV. Inset is the isosurface ( ρ =7 × 10 −3 e Å −3 ) of the decomposed charge density corresponding to the band B in a . Full size image We can integrate the electron density of the localized midgap state ( Fig. 4c ) to obtain the total charge of 3e donated by a single SV, which, as expected, come from the three unsaturated Mo atoms. When n is below a critical density (~10 13 –10 14 cm −2 ), the Fermi level is in the vicinity of gap states and electrons are localized ( Fig. 2b ). As n is above the critical density, the gap states are filled and band-like transport is expected ( Fig. 2a ). This picture naturally explains the metal–insulator transition observed in MoS 2 devices [13] , [31] . We also performed DFT calculations on smaller supercells (4 × 4, 3 × 3 and 2 × 2) corresponding to higher vacancy concentrations. As shown in Supplementary Figs S4–S6 , the defect states are broadened and have a tendency to be more delocalized with the increase of the SV concentration. This is a result of increased interactions between sulphur vacancies in adjacent supercells. We note that the threshold carrier density for the metal–insulator transition in thick (~20 nm) sample [13] was about an order of magnitude lower than predicted by our model, probably due to screening effects and variations of defect density. Evidence of midgap states in MoS 2 was also reported previously [32] . The above analysis makes it logical to interpret the transport data at low carrier densities by hopping mechanism, which has been widely observed in disordered materials [23] , [24] , [33] . At high temperatures, the transport is dominated by nearest-neighbour hopping showing an activated behaviour with T 0 ~300–650 K ( Fig. 2c ). Following Mott’s approach [34] , assuming a constant density of states N μ near the Fermi level, the activation barrier is the energy spacing between nearest sites. Taking T 0 =500 K and a =1.7 nm, , within the range of DFT calculations (considering Gauss broadening, for the midgap state in Fig. 4a ). T 0 was found to decrease with increasing n ( Fig. 2c ). Such trend could be explained by the increase of as the Fermi level approaches the mobility edge. As T decreases, hops over longer distance but with closer energy spacing are more favourable and the transport changes to Mott VRH [34] . According to Tessler et al . [33] , for 2D systems, the electron hopping probability where is localization length. As shown in Fig. 4b , most of the localized electrons are distributed within 6 Å diameter regime surrounding an SV. To further confirm the length scale of , we employed tight-binding calculations and Anderson model (see Methods). Supplementary Fig. S7 gives the correlation between and average conductance G , which is dependent on the Anderson disorder parameter W describing the random potential in the sample (see Supplementary Fig. S8 ). The average conductance was obtained over an ensemble of samples with different configurations of the same disorder strength W . In the localized regime (the low conductance regime), was on the order of few angstroms, which was consistent with the distribution of electron wave function in the DFT calculations. We note that the slight variation of does not affect our conclusions qualitatively, so we use =6 Å in the following discussions. The optimal hopping distance can be obtained by minimizing the right hand side of equation 2, where is the characteristic temperature in equation 1. The cross-over temperature T * is naturally given by R 0 =a (ref. 24 ), which yields . The experimental data is consistent with the hopping model at low electron densities ( T * ~0.15 T 0 at n =10 11 cm −2 ). To account for the discrepancy at high densities ( T * ~0.35 T 0 at n =2.5 × 10 12 cm −2 ), we estimate the Debye screening length ~1.1 nm at 100 K, which becomes comparable to . This results in an increase of due to enhanced screening [35] and accordingly, T * /T 0 . Next we discuss T 1 and its dependence on carrier density and dielectric environment. For the back-gated device, T 1 /T 0 ~90 at n =10 11 cm −2 and gradually decreased to ~20 at n =2.5 × 10 12 cm −2 ( Fig. 2d,e ). The hopping model in equation 3 predicts T 1 /T 0 =69, which again agrees well with experiments at low carrier densities. The decrease of T 1 at high densities could also be explained by enhanced screening [35] . In fact, when the Debye screening length is smaller than (at higher n ), electrons are delocalized, the hopping model is no longer valid. To further test the hopping model, we spin-coated PMMA (dielectric constant ~3.7) after the low temperature measurements and immediately cooled down the device again (see Supplementary Fig. S9 ). We observed an increase of T 1 by a factor of ~5 after PMMA coating, whereas T 0 did not change significantly ( Fig. 2d,e ). Due to the change of dielectric environment, was expected to increase by a factor of ~2. Such screening effect led to a more localized trapping potential and higher T 1 accordingly. We also investigated thicker samples up to tri-layer, all of which showed hopping transport behaviour. In Supplementary Fig. S10 , data from a bi-layer sample are presented. We observed variations of the characteristic temperatures for samples with different thickness. Such variations could be due to sample quality variation, screening by adjacent layers [19] or interlayer coupling [36] , [37] . For thicker samples, we expect that the enhanced screening leads to a higher T * /T 0 . To test such prediction, we fabricated a device on a 4.9-nm-thick sample, corresponding to ~7 layers. The electrical data were summarized in Supplementary Fig. S11 . For n =1–2.5 × 10 12 cm −2 , T * /T 0 is in the range of 0.29–0.54, indeed higher than the single-layer device ( Fig. 2 ). We also observed metallic behaviour above ~250 K, indicating the increasing contribution of bulk transport [17] . As the sample thickness further increases, bulk contribution becomes dominant [19] , and, at some point, a breakdown of the 2D hopping model is expected. In fact, the higher mobility in thicker devices indeed suggested carrier scattering dominated by phonons and long-range Coulomb impurities [17] , [19] . In conclusion, we showed that the charge transport of few-layer MoS 2 in low-carrier-density regime can be explained by hopping through defect-induced localized states. The hopping model was supported by the direct TEM observation of SV, DFT calculations of band structure and tight-binding calculations of localization length. Our study revealed the important role of short-range disorders on the MoS 2 device performance and the need to further improve sample quality by methods such as chemical vapour deposition [38] , [39] . MoS 2 device fabrication and measurement We did micro-cleavage of MoS 2 flakes (SPI supplies) on degenerately doped Si substrates with 300 nm thermal oxide. We used photolithography to pattern source/drain contacts, followed by electron beam evaporation of 40-nm-thick Ti electrodes and lift-off. Ti contacts were used to give low contact resistances [40] . The devices were further annealed at 300°C in a mixture of hydrogen and argon to improve contacts. Electrical measurements were carried out in a close-cycle cryogenic probe station with base pressure ~10 −5 Torr. TEM characterizations of MoS 2 samples MoS 2 samples were exfoliated by micromechanical cleavage techniques from natural MoS 2 bulk crystals (SPI supplies) and transferred to a holy carbon-coated copper TEM grid by the PMMA-based transfer method [41] . To remove the polymer residue on the sample, annealing at 200 °C in a mixture of hydrogen and argon was carried out before TEM. TEM imaging was carried out in an image aberration-corrected TEM (FEI Titan 80–300 operating at 80 kV) and a charge-coupled device camera (2 × 2k, Gatan UltraScanTM 1000) is used for image recording with an exposure time of 1 s. The third-order spherical aberration was set in the range 1–6 μm, and the TEM images were recorded under slightly underfocused. Using a positive value of the third-order spherical aberration, a small defocus yields black atom positions in the TEM images. The electron beam was set to normal imaging conditions with uniform illumination at beam current density~3 A cm −2 . To enhance the visibility of the defects, a Fourier filter was applied to all TEM images. The atomic defects were also visible in the original images, although with lower signal-to-noise ratio (see Supplementary Fig. S12 ). It is noteworthy that long-time electron irradiation at 80 kV could generate SVs due to knock-on damage [28] , [29] . Therefore, after we moved to an area, we limited the exposure time to <30 s (to adjust focus) before imaging. Details of DFT calculations The DFT calculations were carried out using the Vienna ab initio simulation package [42] with projected augmented-wave pseudopotentials [43] and the Perdew–Burke–Ernzerhof exchange and correlation functional [44] . The kinetic energy cutoff for plane wave basis set is 400 eV. All atomic positions were fully relaxed without any symmetry constraint until the Hellmann–Feynman force on each ion and total energy change are <0.01 eV Å −1 and 1 × 10 −4 eV, respectively. The Brillouin zone is sampled by 5 × 5 × 1 and 9 × 9 × 1 k-point meshes within Monkhorst–Pack scheme [44] for geometry optimizations and density of states, respectively. Details of tight-binding calculations The tight-binding method was applied to calculate electronic transport and estimate the localization length of the MoS 2 monolayer. The calculation involves the defect structure created by the SV and a random on-site potential W in the spirit of Anderson model. The disordered system has 5 × 5 supercells (see Supplementary Fig. S3 ). We have adopted the following empirical parameters (all in unit of eV): hopping integral energy t =0.5 describes the bonding between neighbouring Mo and S atoms, on-site potentials of +1 and −1 correspond to the Mo cation and S anion, respectively, on top of that a random on-site potential with a uniform distribution [− W /2, W /2] is added to all lattice sites. For monolayer MoS 2 with W =0 and no SV, the system exhibits a bandgap of 2 eV, close to experimental [4] and other theoretical results [45] . In Anderson model, depends on the random on-site potential W , which is difficult to measure experimentally. To correlate more with experiment, we calculated the conductance of the system under different W . We placed two semi-infinite metallic leads on both ends of the MoS 2 sample and set the on-site energy of the leads to zero to mimic metallic electrodes bridged by the central MoS 2 . The conductance of the system is calculated by using the Green’s function and Landauer formalism [46] , [47] . As expected, we observed the evolution of conductance by varying the disorder strength W , from ballistic, diffusive to the localized regimes (see Supplementary Fig. S8 ). Finally, could be defined as , where L and N c are the sample length and the number of conducting channels, respectively. An increased sample size (like the ones used in experiments) may give much larger conductance at higher energy levels but such size dependence does not exist for electron transport at the Fermi level, which is relevant to our moderate gating voltage. How to cite this article: Qiu, H. et al . Hopping transport through defect-induced localized states in molybdenum disulphide. Nat. Commun. 4:2642 doi: 10.1038/ncomms3642 (2013).